Co-option of a photoperiodic growth-phase transition system during land plant evolution Photoperiodic control of the phase transition from vegetative to reproductive growth is critical for land plants. The GIGANTEA (GI) and FLAVIN-BINDING KELCH REPEAT F-BOX1 (FKF1) protein complex controls this process in angiosperms. However, little is known about how plants evolved this regulatory system. Here, we report that orthologues of GI and FKF1 are present in a basal plant, the liverwort Marchantia polymorpha , and describe the molecular interaction between their products. Knockout of either the GI or FKF1 orthologue completely abolishes the long-day-dependent growth-phase transition in M. polymorpha . Overexpression of either gene promotes growth-phase transition, even under short-day conditions. Introduction of the GI orthologue partially rescues the late-flowering phenotype of the Arabidopsis thaliana gi mutant. Our findings suggest that plants had already acquired the GI-FKF1 system to regulate growth-phase transition when they colonized land, and that this system was co-opted from gametophyte to sporophyte generation during evolution. Perception of day length is the most reliable way for living organisms, including land plants, to predict seasonal changes. Throughout the life cycles of land plants, one of the most important events regulated by day length information is the transition from vegetative phase to reproductive phase. The molecular mechanism of the photoperiodic growth-phase transition has been extensively studied in angiosperms [1] , [2] , [3] . In the long-day plant A. thaliana , GI and FKF1 play essential roles in the regulation of photoperiodic flowering [4] , [5] . GI is a large protein with domains of unknown function. It interacts with FKF1 to form a protein complex in the presence of blue light [4] . The GI-FKF1 complex is involved in the degradation of CYCLING DOF FACTOR1 (CDF1), CDF2, CDF3 and CDF5, which are transcriptional repressors of the flowering gene CONSTANS ( CO ) [6] , [7] . Homologues of GI and FKF1 have been reported in a wide variety of vascular plants from lycophytes to angiosperms [8] . The function of GI in the regulation of photoperiodic flowering has been shown to be common across several angiosperm species [9] , [10] , [11] , [12] , [13] . However, neither GI nor FKF1 orthologues have yet been identified in fully sequenced non-vascular plants, including the moss Physcomitrella patens [8] . Therefore, it has been speculated that the GI and FKF1 genes emerged around the time of the divergence of vascular plants from non-vascular plants [8] . The photoperiodic growth-phase transition operates in diverse plant taxa, from bryophytes to angiosperms [2] , [14] , [15] ; however, underlying molecular mechanisms in non-vascular plants remain unclear. The liverwort M. polymorpha shows a clear photoperiodic growth-phase transition [14] , [16] . Liverworts represent a critical point in the early evolution of land plants, especially the water-to-land transition [17] , [18] . In addition, molecular genetic tools including transformation techniques [19] , [20] , [21] , [22] and strategies for targeted genome modification [23] , [24] have been established for M. polymorpha . Here, we show that the GI-FKF1 complex is present in the gametophyte generation of M. polymorpha , and that it plays an important role in regulating photoperiodic growth-phase transition in this generation. Also, we demonstrate the equivalent functionality of GI between M. polymorpha and A. thaliana . These results give an insight into the evolution of the regulatory mechanism controlling photoperiodic growth-phase in land plants. Identification of GI and FKF1 orthologues in M. polymorpha Under long-day conditions, M. polymorpha undergoes a transition from the vegetative to reproductive phase and initiates the formation of gametangiophores, which contain antheridia or archegonia, at the tips of gametophyte thalli [14] , [16] , [25] , [26] ( Supplementary Fig. 1 ). Exposure to far-red light (FR) is indispensable for this process [19] , suggesting the presence of light-quality- and day-length-dependent regulatory mechanisms in M. polymorpha . Interestingly, and in contrast to the aforementioned information, analysis of genome and transcriptome databases of M. polymorpha revealed single-copy orthologues for GI and FKF1 , designated as MpGI and MpFKF , respectively ( Fig. 1 ). The intron insertion sites in the GI and FKF1 sequences are conserved between M. polymorpha and A. thaliana , with the exception of the first intron insertion sites of GI ( Fig. 1a ). MpGI is predicted to encode 1,187 amino-acid residues, with an estimated molecular mass of 127.5 kDa, thus showing similarity to GI homologues in vascular plants ( Fig. 1b ). MpFKF is predicted to encode 635 amino acids with an estimated molecular mass of 69.5 kDa. The sequence contains a LOV domain, F-box, and six tandem kelch motifs, similar to previously reported for FKF1 and its homologues, ZEITLUPE ( ZTL ) and LOV KELCH PROTEIN2 ( LKP2 ) in A. thaliana [27] , [28] , [29] ( Fig. 1c ). A cysteine residue that is involved in blue light perception via non-covalently binding to a chromophore, flavin mononucleotide (FMN), is conserved between MpFKF and A. thaliana FKF1 (ref. 5 ) ( Fig. 1c ). In a phylogenetic analysis, MpFKF formed a subgroup with an FKF homologue in Selaginella moellendorffii , which was independent from either the ZTL/LKP2 or FKF1 clade in angiosperms ( Fig. 2 ). 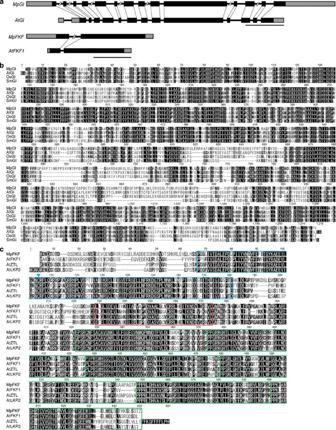Figure 1:Primary structures ofMpGIandMpFKF. (a) Gene structure ofGIandFKF1homologues inM. polymorphaandA. thaliana. Black boxes, grey boxes and black lines indicate exons, untranslated regions and introns, respectively. Scale bar, 1 kb. Introns present inM. polymorphagenes are connected to the corresponding regions inA. thalianagenes by dashed lines. (b,c) Alignment of amino-acid sequences from GI (b) and FKF1 (c) homologues inM. polymorpha,A. thaliana,O. sativaandS. moellendorffii. Identical and similar amino-acid residues are highlighted and shaded, respectively. The conserved cysteine residue involved in FMN binding is indicated by a blue triangle. Blue, red and green open boxes indicate LOV domain, F-box and kelch motifs, respectively. Figure 1: Primary structures of MpGI and MpFKF . ( a ) Gene structure of GI and FKF1 homologues in M. polymorpha and A. thaliana . Black boxes, grey boxes and black lines indicate exons, untranslated regions and introns, respectively. Scale bar, 1 kb. Introns present in M. polymorpha genes are connected to the corresponding regions in A. thaliana genes by dashed lines. ( b , c ) Alignment of amino-acid sequences from GI ( b ) and FKF1 ( c ) homologues in M. polymorpha , A. thaliana , O. sativa and S. moellendorffii . Identical and similar amino-acid residues are highlighted and shaded, respectively. The conserved cysteine residue involved in FMN binding is indicated by a blue triangle. Blue, red and green open boxes indicate LOV domain, F-box and kelch motifs, respectively. 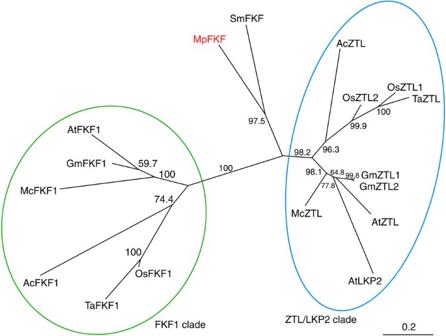Figure 2: Phylogenetic analysis of MpFKF. An unrooted maximum-likelihood phylogenetic tree was estimated using amino-acid sequences of FKF/ZTL/LKP2 homologues. Protein sequences used for the analysis were fromA. thaliana(AtFKF1, AtZTL, and AtLKP2),O. sativa(OsFKF1, OsZTL1 and OsZTL2),Glycine max(GmFKF1, GmZTL1 and GmZTL2),Triticum aestivum(TaFKF1 and TaZTL),Allium cepa(AcFKF1 and AcZTL),Mesembryanthemum crystallinum(McFKF1 and McZTL) andS. moellendorffii(SmFKF). The clade that consists of FKF homologues is marked with green, and the clade consisting of LKP2/ZTL homologues with blue. Scale bar, evolutionary distance in substitutions per residue. Numbers, bootstrap probabilities. Full size image Figure 2: Phylogenetic analysis of MpFKF. An unrooted maximum-likelihood phylogenetic tree was estimated using amino-acid sequences of FKF/ZTL/LKP2 homologues. Protein sequences used for the analysis were from A. thaliana (AtFKF1, AtZTL, and AtLKP2), O. sativa (OsFKF1, OsZTL1 and OsZTL2), Glycine max (GmFKF1, GmZTL1 and GmZTL2), Triticum aestivum (TaFKF1 and TaZTL), Allium cepa (AcFKF1 and AcZTL), Mesembryanthemum crystallinum (McFKF1 and McZTL) and S. moellendorffii (SmFKF). The clade that consists of FKF homologues is marked with green, and the clade consisting of LKP2/ZTL homologues with blue. Scale bar, evolutionary distance in substitutions per residue. Numbers, bootstrap probabilities. Full size image In A. thaliana , the transcription of GI and FKF1 genes is regulated by the circadian clock [27] , [30] , [31] . Similarly, in mature thalli grown under 12-h-light/12-h-dark cycles, MpGI and MpFKF showed diurnal expression patterns, with phase peaks occurring around dusk ( Fig. 3a,b ). Furthermore, the rhythmic expression of MpGI and MpFKF persisted after the transition to constant light or dark conditions, suggesting that the expression of MpGI and MpFKF is regulated by the circadian clock ( Fig. 3c–f ). 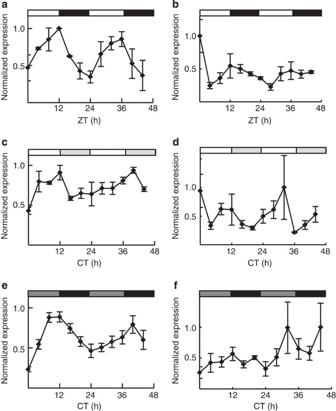Figure 3:Circadian expression ofMpGIandMpFKFinM. polymorpha. (a–f) Transcript accumulation profiles ofMpGI(a,c,e) andMpFKF(b,d,f) monitored under a 12-h-light/12-h-dark cycle (a,b), constant light (c,d) and constant dark (e,f) conditions. Bars above the traces represent light conditions; open, filled, lightly shaded and darkly shaded bars represent day, night, subjective night and subjective day, respectively. ZT, Zeitgeber time; CT, circadian time (time after the transfer from light-dark cycles to constant conditions). Error bars, s.e.m.;n=3. Figure 3: Circadian expression of MpGI and MpFKF in M. polymorpha. ( a – f ) Transcript accumulation profiles of MpGI ( a , c , e ) and MpFKF ( b , d , f ) monitored under a 12-h-light/12-h-dark cycle ( a , b ), constant light ( c , d ) and constant dark ( e , f ) conditions. Bars above the traces represent light conditions; open, filled, lightly shaded and darkly shaded bars represent day, night, subjective night and subjective day, respectively. ZT, Zeitgeber time; CT, circadian time (time after the transfer from light-dark cycles to constant conditions). Error bars, s.e.m. ; n =3. Full size image Interaction between MpGI and MpFKF We next examined complex formation between MpGI and MpFKF. Yeast two-hybrid analysis indicated an interaction between full-length proteins of MpGI and MpFKF ( Fig. 4a ). Truncation analysis revealed that the 392 amino-acid residues of the MpGI N terminus and the LOV domain of MpFKF were sufficient for the interaction ( Fig. 4a ). Coimmunoprecipitation of 3 × FLAG-tagged MpGI with 4 × myc-tagged MpFKF in transgenic plants suggests that the interaction between MpGI and MpFKF also occurs in vivo ( Fig. 4b ). Spatial expression analysis of MpGI and MpFKF , using plants expressing the GUS reporter gene under the control of their promoter sequences, revealed overlapping GUS staining, which was observed continuously from the apical notch region to the midrib of mature thalli ( Fig. 4c,d ). These results suggest that the MpGI and MpFKF protein complex accumulates in the gametophyte of M. polymorpha . 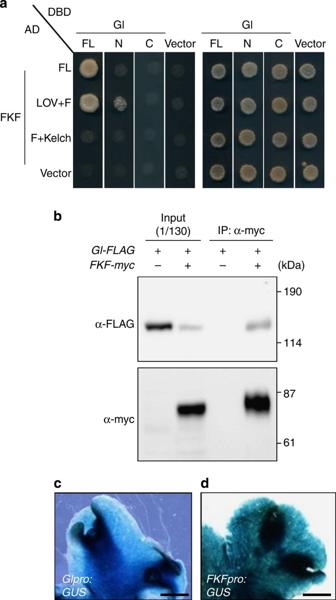Figure 4: Interactions and spatial expression of MpGI and MpFKF. (a) Yeast two-hybrid analysis. Full-length (FL) or truncated MpGI and MpFKF fused to the DNA-binding domain (DBD) or the activation domain (AD) of Gal4 were tested under selective (−WLH, left) and non-selective (−WL, right) conditions. For MpGI, N and C indicate the amino-acid residues 1–392 and 383–1,187, respectively. For MpFKF, F and Kelch indicate F-box and kelch-repeat domains, respectively. (b) Co-immunoprecipitation of GI-FLAG and FKF-myc from the extracts of plants overexpressing MpGI-FLAG only or both MpGI-FLAG and MpFKF-myc. Anti-FLAG (α-FLAG) and anti-c-Myc (α-myc) antibodies were used to detect MpGI-FLAG and MpFKF-myc, respectively, by western blotting. (c,d) GUS staining images from 10-day-old plants harbouringMpGIpro:GUS(c) orMpFKFpro:GUS(d). Scale bar, 1 mm. Figure 4: Interactions and spatial expression of MpGI and MpFKF. ( a ) Yeast two-hybrid analysis. Full-length (FL) or truncated MpGI and MpFKF fused to the DNA-binding domain (DBD) or the activation domain (AD) of Gal4 were tested under selective (−WLH, left) and non-selective (−WL, right) conditions. For MpGI, N and C indicate the amino-acid residues 1–392 and 383–1,187, respectively. For MpFKF, F and Kelch indicate F-box and kelch-repeat domains, respectively. ( b ) Co-immunoprecipitation of GI-FLAG and FKF-myc from the extracts of plants overexpressing MpGI-FLAG only or both MpGI-FLAG and MpFKF-myc. Anti-FLAG (α-FLAG) and anti-c-Myc (α-myc) antibodies were used to detect MpGI-FLAG and MpFKF-myc, respectively, by western blotting. ( c , d ) GUS staining images from 10-day-old plants harbouring MpGIpro:GUS ( c ) or MpFKFpro:GUS ( d ). Scale bar, 1 mm. Full size image Essential role of MpGI and MpFKF in growth-phase transition To investigate the physiological function of the MpGI-MpFKF complex in M. polymorpha , we generated knockout mutants of both MpGI and MpFKF using a homologous recombination-mediated gene targeting strategy [23] . Disruption of these genes was performed by replacing the second exon of MpGI and a 264-bp region of MpFKF , including the conserved FMN-binding domain, with a hygromycin-resistant marker ( Supplementary Fig. 2a,b ). Genomic PCR analysis confirmed the homologous recombination events on the MpGI and MpFKF loci, in the gi ko and fkf ko lines, respectively ( Supplementary Fig. 2c,d ). RT-PCR analysis revealed that MpGI and MpFKF gene expression was undetectable in these lines ( Supplementary Fig. 2e,f ). Ten-day-old wild-type and knockout thalli grown from gemmae under constant light conditions were subjected to long-day conditions supplemented with FR. Under these conditions, individual wild-type plants formed the first visible gametangiophore within 20 days, whereas neither gi ko nor fkf ko plants formed any gametangiophores after 60 days, indicative of a failure of the growth-phase transition in the knockout lines ( Fig. 5a,b ). These defects were rescued by introducing the genomic fragment of MpGI or MpFKF ( Fig. 5a,b , and Supplementary Fig. 2e,f ). This indicates that the MpGI and MpFKF genes are required for growth-phase transition under long-day conditions. Given that MpGI could interact with MpFKF in vivo , and that a single disruption of MpGI or MpFKF caused equally severe defects in the growth-phase transition without mutually affecting their transcription ( Supplementary Fig. 2g ), these observations suggest that formation of the MpGI and MpFKF complex is critical for growth-phase transition in M. polymorpha . 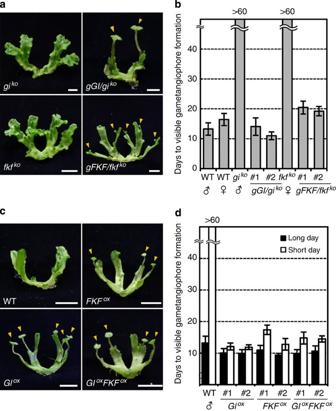Figure 5:Effects of disruption and overexpression ofMpGIandMpFKFon the growth-phase transition ofM. polymorpha. (a,b) Timing of gametangiophore formation in wild-type plants, knockout mutants ofMpGI(giko, male) andMpFKF(fkfko, female) and their complementation lines (gGI/gikoandgFKF/fkfko; two lines for each). Plants were grown from gemmae under long-day conditions. (c,d) Timing of gametangiophore formation in wild-type plants and lines overexpressingMpGI(GIox),MpFKF(FKFox) or both (GIoxFKFox). Plants were grown from gemmae under long- and short-day conditions. Photographs of 35-day-old plants (a,c) and days to the first visible gametangiophore formation (b,d) are shown. Arrowheads indicate gametangiophores. WT, wild type. Scale bar, 10 mm. Error bars, s.d.;n>15. Figure 5: Effects of disruption and overexpression of MpGI and MpFKF on the growth-phase transition of M. polymorpha . ( a , b ) Timing of gametangiophore formation in wild-type plants, knockout mutants of MpGI ( gi ko , male) and MpFKF ( fkf ko , female) and their complementation lines ( gGI/gi ko and gFKF/fkf ko ; two lines for each). Plants were grown from gemmae under long-day conditions. ( c , d ) Timing of gametangiophore formation in wild-type plants and lines overexpressing MpGI ( GI ox ), MpFKF ( FKF ox ) or both ( GI ox FKF ox ). Plants were grown from gemmae under long- and short-day conditions. Photographs of 35-day-old plants ( a , c ) and days to the first visible gametangiophore formation ( b , d ) are shown. Arrowheads indicate gametangiophores. WT, wild type. Scale bar, 10 mm. Error bars, s.d. ; n >15. Full size image Effect of overexpression of MpGI or MpFKF on photoperiodism In A. thaliana , simultaneous overexpression of GI and FKF1 increases the amount of GI-FKF1 complex and eliminates photoperiodicity to promote flowering under short-day conditions [4] . To examine whether overexpression of MpGI and MpFKF alters photoperiodic growth-phase transition in M. polymorpha , we generated overexpression lines of MpGI-FLAG or MpFKF-myc under the control of an M. polymorpha ELONGATION FACTOR1-α (MpEF) promoter [32] . In wild-type plants, gametangiophore formation is delayed under short-day conditions ( Fig. 5d and Supplementary Fig. 1 ), whereas the number of days required for gametangiophore formation in the overexpression lines of either gene was significantly shortened and was comparable to those of wild-type plants grown under long-day conditions ( Fig. 5c,d ). In addition, the growth-phase transition of these overexpression lines under long-day conditions was slightly promoted ( Fig. 5d ). Simultaneous overexpression of MpGI-FLAG and MpFKF-myc did not enhance the phenotype caused by single-gene over expression, suggesting that MpGI and MpFKF may act genetically in the same pathway. These results suggest that overexpression of MpGI or MpFKF could increase the amount of MpGI-MpFKF complex and promote the growth-phase transition regardless of photoperiod. Overexpression of only MpGI-FLAG in the fkf ko background or only MpFKF-myc in the gi ko background did not promote growth-phase transition under short-day conditions within 3 weeks. In contrast, all overexpression lines in the wild-type background formed gametangiophores within 3 weeks ( Fig. 5d ). These findings supported our hypothesis that MpGI and MpFKF co-require each other and function as a complex. It is noteworthy that under white light conditions without FR supplementation, no gametangiophore formation was observed by day 60 in any of the overexpression lines. Therefore, the MpGI- and MpFKF-mediated photoperiodic pathway is likely to act independently of the light-quality-dependent pathway to regulate growth-phase transition in M. polymorpha . Complementation of Arabidopsis gi with MpGI Our findings showed that the regulatory system of photoperiodic growth-phase transition mediated by GI-FKF1 is present in the gametophyte of liverwort. To examine whether MpGI is functionally equivalent to angiosperm GI and able to function in the regulation of flowering, we introduced MpGI into an A. thaliana gi mutant [30] , [31] . Expression of MpGI under the control of the AtGI promoter partially complemented the late-flowering phenotype of the A. thaliana gi mutant ( Fig. 6 ), suggesting that the MpGI gene has the potential to act as a regulator of flowering. 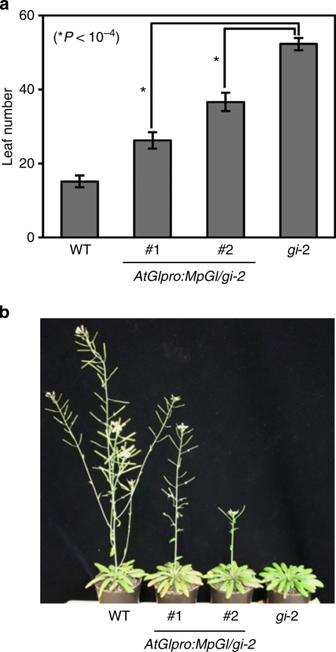Figure 6:Genetic complementation of theA. thaliana gimutantbyMpGI. (a) Rosette leaf numbers of wild-typeA. thaliana(Columbia-0),gi-2, andgi-2harbouring anAtGIpro:MpGIconstruct, at the time of bolting under long-day conditions. *P<10−4. Error bars, s.d.;n>10.P-values were determined using unpaired Student’st-test. (b) Representative individuals of wild type,gi-2,andAtGIpro:MpGI/gi-2at 45 days after germination. WT, wild type. Figure 6: Genetic complementation of the A. thaliana gi mutant by MpGI. ( a ) Rosette leaf numbers of wild-type A. thaliana (Columbia-0), gi-2 , and gi-2 harbouring an AtGIpro:MpGI construct, at the time of bolting under long-day conditions. * P <10 −4 . Error bars, s.d. ; n >10. P -values were determined using unpaired Student’s t -test. ( b ) Representative individuals of wild type, gi-2, and AtGIpro:MpGI/gi-2 at 45 days after germination. WT, wild type. Full size image In this study, we demonstrated that both M. polymorpha and A. thaliana use the GI-FKF1 system to regulate photoperiodic growth-phase transition. This suggests that the molecular mechanisms regulating gametangiophore formation in the liverwort are equivalent to those involved in flowering in angiosperms. In A. thaliana , the GI-FKF1 complex directly degrades CDF1 and regulates flowering time via transcriptional regulation of the flowering genes CO and FLOWERING LOCUS T ( FT ) [1] . Although these genes that regulate flowering are widely conserved in angiosperms [2] , a previous report on CO homologues in P. patens showed that they are more closely related to CO-like genes, AtCOL3/AtCOL4/AtCOL5, which form a distinct group from CO [33] . Also, the presence of FT is controversial. In the phosphatidylethanolamine-binding protein (PEBP) gene family, the family to which FT and TERMINAL FLOWER1 ( TFL1 ) belong [34] , [35] , the genes in the FT/TFL1 subfamily were suggested to have arisen in seed plants, since they are absent from the genomes of P. patens and S. moellendorffii [36] . Identification of the growth-phase transition regulators that are downstream of the MpGI-MpFKF complex will greatly advance our understanding of how photoperiodic growth-phase regulation mechanisms evolved in land plants. The presence of the GI-FKF1 complex in the liverwort lineage strongly suggests that this system had already been acquired in the common ancestor of land plants. Sequencing of the genomes of species in the Charophyceae, a class with a sister relationship to land plants [17] , as well as comparative genomic approaches will be required to further understand the evolutionary novelty of the GI-FKF1 system during the course of green plant evolution. Interestingly, the GI-FKF1 system functions in the gametophyte generation in M. polymorpha , whereas it functions in the sporophyte generation in A. thaliana . These facts imply that, during the course of land plant evolution, the GI-FKF1 system that evolved to regulate reproductive phase transition in the gametophyte generation in basal land plants was co-opted to regulate that in the sporophyte generation in vascular plants. Plant material and growth conditions Male and female accessions of M. polymorpha , Takaragaike-1 (Tak-1) and Takaragaike-2 (Tak-2), respectively [20] were used as the wild type. Plants were cultured axenically on half-strength Gamborg’s B5 medium [37] containing 1% sucrose and 1.3% agar, under a 50–60 μmol m −2 s −1 continuous white cold cathode fluorescent lamp (CCFL; OPT-40C-N-L, Optrom) at 22 °C, unless otherwise defined. For analysis of growth-phase transition, gametangiophores were induced in growth chambers (LH-80CCFL-6CT, NKSystem) under long-day (16-h-light/8-h-dark) or short-day (8-h-light/16-h-dark) conditions using 40–60 μmol m −2 s −1 CCFL supplemented with 20–30 μmol m −2 s −1 FR light-emitting diodes (VBL-TFL600-IR730*, Valore; peak emission at 733 nm, with a full width at half maximum of 27 nm) at 22 °C. Sequence retrieval and phylogenetic analysis The search for M. polymorpha GI and FKF1 gene homologues was performed using the transcriptome and genome databases from the M. polymorpha on-going Joint Genome Institute genome-sequencing project ( http://www.jgi.doe.gov/ ). Protein alignments were constructed using MUSCLE alignment implemented in the Geneious 6.1.6 software package (Biomatters; http://www.geneious.com ) at the default parameters, and an unrooted maximum-likelihood phylogenetic tree constructed using PhyML program ver. 2.2.0 (ref. 38 ) implemented in the Geneious software, using the LG model and four categories of rate substitution. Tree topology, branch length and substitution rates were optimized, and the tree topology was searched using the nearest-neighbour interchange method. Bootstrap values were computed from 1,000 trials. The sequences used for the protein alignment of GI homologues were AtGI (ABP96497) from A. thaliana , OsGI (Os01g0182600) from Oryza sativa and SmGI (XP_002961231) from S. moellendorffii. The sequences used in the phylogenetic tree of FKF1/ZTL/LKP2 were as follows: AtFKF1 (AAF32298), AtZTL (NP_001154783), AtLKP2 (NP_849983) from A. thaliana ; OsFKF1 (Os11g0547000), OsZTL1 (Os02g0150800), OsZTL2 (Os06g0694000) from O. sativa; GmFKF1 (NP_001235886), GmZTL1 (NP_001235856), GmZTL2 (NP_001235871) from Glycine max ; TaFKF1 (ABL11478), TaZTL (ABR14627) from Triticum aestivum ; AcFKF1 (ACT22762), AcZTL (ACT22763) from Allium cepa ; McFKF1 (AAQ73528), McZTL (AAQ73527) from Mesembryanthemum crystallinum ; and SmFKF (XP_002974336) from S. moellendorffii. Plasmid construction To generate the MpGI -targeting vector, 3.5-kb homologous arms were amplified from Tak-1 genomic DNA by PCR using KOD FX Neo (Toyobo) with the primer pairs: forward 5′-CTAAGGTAGCGATTAATGCAGGAATAGTAGAGATCATGAAGG-3′, reverse 5′-CCGGGCAAGCTTTTAATCGTGAAACGATCCCAAATCT-3′ (for the 5′ side); and forward 5′-AACACTAGTGGCGCGAGCCAAAGAACCGTATCGAA-3′, reverse 5′-TTATCCCTAGGCGCGTGGCATTCCATTCTATGCTG-3′ (for the 3′ side). The PCR-amplified fragments of the 5′ end and 3′ end were cloned into the PacI site and AscI sites of pJHY-TMp1 (ref. 23 ), respectively, using an In-Fusion HD cloning kit (Clontech). The MpFKF -targeting vector was designed in the reverse direction to that of MpGI . 6-kb homologous arms that were amplified using the primer pairs: forward 5′-TTATCCCTAGGCGCGCACACTCCGTGCAATCTCAA-3′, reverse 5′-TAAACTAGTGGCGCGCCACAACGATCCTACCACATC-3′ (for the 5′ side), and forward 5′-GCCCGGGCAAGCTTAACCATGGAAGGACTCACTGC-3′, reverse 5′-CTAAGGTAGCGATTAAGTTCGGACAGCTTCCTTCA-3′ (for the 3′ side), and cloned into the AscI site and PacI site of pJHY-TMp1 (ref. 23 ), respectively. The resultant targeting vectors were introduced into F 1 sporelings of M. polymorpha derived from crosses between Tak-1 and Tak-2, as described previously [20] . Screening for gene-targeted lines was performed by genomic PCR as described previously [23] . Gene-specific primers used in the screening are illustrated in Supplementary Fig. 2a,b and Supplementary Table 1 . For the complementation test of gi ko and fkf ko , genomic fragment including entire regions of MpGI and MpFKF was amplified from Tak-1 genomic DNA by PCR using KOD Plus Neo (Toyobo) with the primer pairs: forward 5′-CACCGCTATTCTTCACGCCGAAA-3′, reverse 5′-TCCCCCTTTATTGTTGAACT-3′ (for MpGI ), and forward 5′-CACCTGACCGTTTAATTCATTGTGGA-3′, reverse 5′-GATGGTTTCCCGTACAGGTG-3′ (for MpFKF ), and cloned into pENTR/D-TOPO (Life Technologies). These were used to generate binary plasmids harbouring MpGIpro:gMpGI or MpFKFpro:gMpFKF. The resultant plasmids were introduced into corresponding knockout mutants, gi ko or fkf ko , as described previously [21] . To construct MpGIpro:GUS and MpFKFpro:GUS , a 4,573-bp fragment of MpGI , and a 5,082-bp fragment of MpFKF , as measured from their predicted start codons, were amplified from Tak-1 genomic DNA by PCR using KOD Plus Neo with the primer pairs: forward 5′-CACCAGATTTTAGGTTGACTCG-3′, reverse 5′-GGGAAATGACATAGGGCCAA-3′ (for MpGI ), and forward 5′-CACCTGACCGTTTAATTCATTGTGGA-3′, reverse 5′-ACCCAAGGACATATCCGAGT-3′ (for MpFKF ), respectively. Each fragment was cloned into pENTR/D-TOPO and used to generate binary plasmids harbouring MpGIpro:GUS and MpFKFpro:GUS , which were introduced into F 1 sporelings generated from Tak-1 and Tak-2 (ref. 20 ). To generate overexpression lines of MpGI and MpFKF , full-length cDNA of MpGI and MpFKF was amplified using the primer pairs: forward 5′-CACCATGTCATTTCCCGGGCAGAA-3′, reverse 5′-GACAGGAATCGGGCAGC-3′ (for MpGI ), and forward 5′-CACCATGGATTGGGATACAGATACCG-3′, reverse 5′-GGTGCTAGACAGACTCTTATGTGTTA-3′ (for MpFKF ). These were fused with 3xFLAG or 4xmyc sequences to generate binary plasmids harbouring MpEFpro:MpGI-3xFLAG and MpEFpro:MpFKF-4xmyc . These overexpression constructs were introduced into cut thalli of Tak-1 as described previously [21] . Transformants, after two cycles of transplantation of gemmae, were used for the remainder of the experiments. Total RNA isolation and cDNA synthesis Tak-1 gemmae were grown under constant light for 9 days, followed by a 12-h-light/12-h-dark cycle for 6 days. From day 16, plants were harvested and immediately frozen in liquid nitrogen at 4-h intervals over 2 days under specific light conditions described in the text for each experiment. The frozen samples were ground into a frozen powder by shaking for 5 min with 6-mm stainless beads in collection tubes using a ShakeMaster (BMS-12-NA, BioMedicalScience). Total RNA was extracted from the powder using TRIzol (Life Technologies) and treated with RQ1 RNase-Free DNase (Promega). For each sample, 4 μg RNA was reverse transcribed to cDNA using random hexamer primers and ReverTra Ace (Toyobo), following the manufacturer's instructions. Quantitative RT–PCR analysis cDNA samples were diluted 1:4 and amplified with the CFX96 Real-Time PCR Detection System (Bio-Rad) using SYBR Green I Nucleic Acid Gel Stain (Lonza) to monitor dsDNA synthesis. Primer sequences and their optimal melting temperatures are listed in Supplementary Table 1 . The three-step PCR cycling program was as follows: 95 °C for 2 min, followed by 40 cycles at 95 °C for 10 s, melting temperature for 15 s and 72 °C extension for 15 s. Melt-curve analysis was performed to ensure specificity of the products. Each cDNA sample was run at least in duplicate. PCR efficiencies were calculated using the software CFX Manager (Bio-Rad) in accordance with the manufacturer’s instructions. Raw expression data were normalized using MpEF expression data, and peak levels were set to 1. The relative expression values of each gene were calculated to show the average±s.e. of mean of three biologically independent trials. Expression of the MpEF reference gene showed constant patterns, without circadian rhythmicity, over all sample time points (data not shown). All primers used for the analysis are listed in Supplementary Table 1 . Co-immunoprecipitation experiments Plants were grown under constant light conditions for 10 days, transferred to FR-supplemented long-day conditions for a further 7 days and harvested at ZT12 of day 18 for use in the experiments. Approximately 500 mg of plants were harvested, frozen in liquid nitrogen and ground into a frozen powder. The protein was extracted in 1 ml of ice-cold IP buffer (50 mM Tris-HCl pH 7.4, 5 mM EDTA, 50 mM NaCl, 1 mM dithiothreitol, 0.1% (v/v) Triton X-100, 10% (v/v) glycerol, 50 μM MG-132 and cOmplete protease inhibitor (Roche)). After centrifugation at 3,500 g for 2 min and 16,400 g for 10 min to remove cell debris, the supernatant containing approximately 5 mg of total protein was mixed with 50 μl of magnetic beads conjugated to an anti-myc antibody (Miltenyi Biotech) and then incubated on ice for 30 min. The mixtures were applied to μColumns (Miltenyi Biotech) in a magnetic field. After 10 washes with 200 μl of IP buffer and one rinse with 150 μl of Wash Buffer 2 (Miltenyi Biotech), proteins were eluted using 90 μl of 2 × sample buffer (60 mM Tris-HCl pH 6.8, 5% sodium dodecyl sulphate (SDS), 20% (v/v) glycerol, and 10% (v/v) 2-mercaptoethanol) to obtain the bound fraction. The immunoprecipitates were then subjected to immunoblot analysis. Immunoblot analysis Proteins were size fractionated using 8% SDS polyacrylamide gel electrophoresis, followed by protein gel blot analysis using a 1:10,000 dilution of anti-FLAG M2 IgG antibody (F1804, Sigma-Aldrich) and a 1:500 dilution of anti-c-Myc IgG antibody (014-21901, Wako Pure Chemical Industries). A 1:10,000 dilution of the horseradish peroxidase-linked anti-mouse IgG antibody (NA931, GE Healthcare) was used as a secondary antibody. Protein blots were visualized using the horseradish peroxidase-based ECL Plus reagent (GE Healthcare) with an Image Quant LAS 4010 biomolecular imager (GE Healthcare). Yeast two-hybrid analysis The GAL4-based yeast two-hybrid system (Matchmaker Gold Yeast Two-Hybrid System, Clontech) was used for detecting protein–protein interactions. Full-length, N-terminal half (amino acids 1–392) and C-terminal half (amino acids 383–1,187) MpGI cDNAs were PCR-amplified and subcloned into the EcoRI-SalI site of pGBKT7 (Clontech). Truncated cDNA clones of MpFKF containing full length, LOV domain+F-box domain (amino acids 1–291) and F-box domain+Kelch repeats (181–635) were PCR amplified and subcloned into the NdeI-BamHI site of pGADT7 (Clontech). After the sequences were confirmed, the plasmids were transformed into the yeast strain AH109 and transformants selected on SD−WL medium. The resulting colonies were cultured in SD−WL liquid medium and then serially diluted in distilled water before being spotted onto SD−WL and SD−WLH plates to analyse the interaction. pGBKT7 and pGADT7 plasmids were used as negative controls for yeast two-hybrid analysis. After a 2- to 3-day-incubation at 28 °C, the plates were photographed. The experiments were repeated three times with similar results. The gene-specific primer sets used for the generation of each construct are given in Supplementary Table 1 . Transformation of MpGI into an A. thaliana gi mutant The upstream regions of AtGI including the promoter and 5′UTR (2,106 bp) and the full-length cDNA of MpGI were amplified by PCR with the primer pairs: forward 5′-CACCTGCCTACAATTTGAGAATACGCC-3′, reverse 5′-TTCTGCCCGGGAAATGACATCCAGGAACCGAAACTAAACCCCAAC-3′ for the upstream regions of AtGI , and forward 5′-GGTTTAGTTTCGGTTCCTGGATGTCATTTCCCGGGCAGAAATGGC-3′ and reverse 5′-TTAGACAGGAATCGGGCAGC-3′ for MpGI cDNA. The PCR products were then subjected to PCR using the primer pairs: forward 5′-CACCTGCCTACAATTTGAGAATACGCC-3′ and reverse 5′-TTAGACAGGAATCGGGCAGC-3′ to generate the AtGIpro:MpGI fused sequence. The resultant fragment was introduced into pGWB1 (ref. 39 ) to generate the AtGIpro:MpGI binary plasmid. pGWB1 were kindly provided by T. Nakagawa (Shimane University). The construct was introduced into the A. thaliana gi-2 mutant using the floral dip method [40] . Transgenic lines that possessed a single copy of the AtGIpro:MpGI construct in gi-2 were used for further analysis. For flowering phenotype analysis, plants were grown on soil in growth chambers (LH300, NKSystem) under 16-h-light/8-h-dark conditions with an illumination rate of 90 to 110 μmol m −2 s −1 of white fluorescent light (FL40SSEX-N/37-HG, NEC Lighting) at 22 °C. The Columbia-0 accession was used as the wild type. Flowering time was measured by counting the number of rosette leaves upon bolting. Histochemical GUS staining The MpGIpro:GUS- and MpFKFpro:GUS- expressing plants were grown on half-strength B5 agar plates containing 1% sucrose for 10 days under continuous light. Histochemical GUS staining was performed as described previously [41] . The staining patterns of GUS activity from more than 10 individual lines were analysed. Representative patterns are shown in Fig. 4 . Accession codes: The sequence of the MpGI and MpFKF genes are available in DDBJ (accession numbers AB872959 for MpGI and AB872960 for MpFKF ). How to cite this article: Kubota, A. et al. Co-option of a photoperiodic growth-phase transition system during land plant evolution. Nat. Commun. 5:3668 doi: 10.1038/ncomms4668 (2014).